A submicron plasmonic dichroic splitter Spectral imaging and sensing techniques, new solar cell designs and wavelength-division multiplexing in optical communication rely on structures that collect and sort photons by wavelength. The strong push for chip-scale integration of such optical components has necessitated ultracompact, planar structures, and fomented great interest in identifying the smallest possible devices. Consequently, novel micro-ring, photonic crystal and plasmonic solutions have emerged. Meanwhile, the optical coupling of subwavelength plasmonic structures supporting a very limited number of modes has also enabled new functionalities, including Fano resonances and structural electromagnetically-induced transparency. Here we show how two similarly sized subwavelength metal grooves can form an ultracompact submicron plasmonic dichroic splitter. Each groove supports just two electromagnetic modes of opposite symmetry that allows independent control of how a groove collects free-space photons and directs surface plasmon polaritons. These results show how the symmetry of electromagnetic modes can be exploited to build compact optical components. Recently there has been much theoretical and experimental research dedicated to miniaturizing optical devices. Broad fundamental limits have been identified that constrain the size of a device, given its general function, shape and range of dielectric constants [1] . The specific goal of chip-scale integration has led to many planar photonic crystal and plasmonic designs such as a compact mode separator [2] and photon sorters [3] , [4] . The push for miniaturization has also created a need to use very small, subwavelength optical scatterers that support just a few electromagnetic modes. Coupling such scatterers together has led to new plasmonic functionalities such as Fano resonances [5] , [6] and structural electromagnetically-induced transparency [7] . Patterned metal films constitute a convenient platform for controlling the flow of light in the form of surface plasmon polaritons (SPPs) and for converting such waves to and from photons. They are particularly effective at controlling visible and near-infrared light as SPPs in this frequency regime are tightly confined to the metal surface and interact strongly with nanoscale perturbations in an otherwise smooth metal film. These essentially planar structures are easily fabricated by thin film deposition and liftoff, etching or ion-milling techniques. This has resulted in a myriad of exciting physical phenomena and applications, including extraordinary optical transmission [8] , [9] , enhanced photodetection [10] , collimated light emission [11] , [12] , subwavelength lithography [13] and microfluidic biosensing [14] . The response of various nanopatterns can be approximated by considering how SPPs propagate along the surface and undergo multiple scattering between individual patterned elements (for example, holes, grooves and slits) [9] , [15] . With this in mind, we were able to design and realize a submicron plasmonic dichroic splitter. Through first simulating the single-scattering events of one groove, we show that the interference of two groove modes allow independent control of how the groove generates and directs surface plasmons. Utilizing this behaviour, we then numerically designed a pair of grooves for dichroic splitting. Finally, grooves were fabricated through focused ion beam milling (FIB), and optical measurement successfully demonstrated a dichroic response with a splitting ratio of 3:1 at shorter wavelengths reversing to 1:2 at longer wavelengths. Our ultracompact dichroic splitter represents another important advance for optical miniaturization through plasmonics. 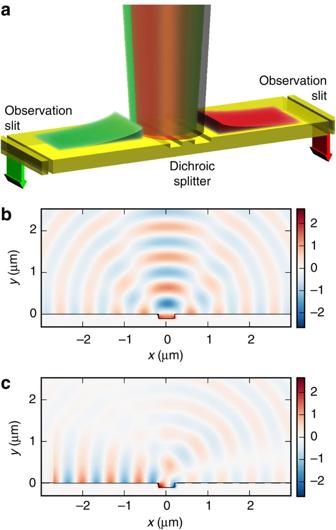Figure 1: Interplay between two mode symmetries enables new chip-scale functionalities. (a) Illustration of the proposed submicron plasmonic dichroic splitter consisting of two grooves of slightly different width. The two-groove structure launches SPPs preferentially to the left or right depending on the wavelength of the incident free-space beam. Off to the side, two equidistant slits cut through the metal film reconvert the launched SPPs back into free-space photons and enable far-field observation. The ability of this structure to efficiently sort photons based on wavelength relies on the fact that the relatively wide (few 100 nm) grooves in the splitter support two modes of different symmetry. As a result, these two modes couple very differently to incident free-space photons and SPPs, as illustrated inbandc. (b) A vertically incident Gaussian beam of transverse magnetic photons only excites SPPs through the fundamental groove mode, which exhibits a symmetric magnetic field about the groove centre. (c) A SPP incident from the left is strongly scattered by the second groove mode, which exhibits an anti-symmetric magnetic field about the groove centre. The simulations were performed at a wavelength of 700 nm for a 380 nm wide and 110-nm-deep groove in Au. The real part of the magnetic field is plotted inbandcwhen its magnitude is maximal within the groove. The magnetic field is directed out of the plane along the length of the groove. Proposed plasmonic dichroic splitter A schematic view of our plasmonic dichroic splitter is shown in Figure 1a . Here photons normally incident on the dichroic splitter are converted to surface plasmons travelling to the left or right depending on the wavelength and then extracted through observation slits for the experiment. Below, we first start with the conceptual design of the dichroic splitter then move to the experimental data. Figure 1: Interplay between two mode symmetries enables new chip-scale functionalities. ( a ) Illustration of the proposed submicron plasmonic dichroic splitter consisting of two grooves of slightly different width. The two-groove structure launches SPPs preferentially to the left or right depending on the wavelength of the incident free-space beam. Off to the side, two equidistant slits cut through the metal film reconvert the launched SPPs back into free-space photons and enable far-field observation. The ability of this structure to efficiently sort photons based on wavelength relies on the fact that the relatively wide (few 100 nm) grooves in the splitter support two modes of different symmetry. As a result, these two modes couple very differently to incident free-space photons and SPPs, as illustrated in b and c . ( b ) A vertically incident Gaussian beam of transverse magnetic photons only excites SPPs through the fundamental groove mode, which exhibits a symmetric magnetic field about the groove centre. ( c ) A SPP incident from the left is strongly scattered by the second groove mode, which exhibits an anti-symmetric magnetic field about the groove centre. The simulations were performed at a wavelength of 700 nm for a 380 nm wide and 110-nm-deep groove in Au. The real part of the magnetic field is plotted in b and c when its magnitude is maximal within the groove. The magnetic field is directed out of the plane along the length of the groove. Full size image Single-groove scattering Depending on their width, narrow rectangular grooves support one or two gap plasmon modes that govern their light scattering behaviour [16] , [17] , [18] . A groove can couple free-space photons onto the metal surface in the form of single-interface SPPs and scatter these SPPs in-plane. Figure 1b shows how SPPs can be generated by top-illuminating a groove with light of a transverse magnetic polarization. Because of symmetry, the vertically incident photons can only couple to the fundamental groove mode for which the magnetic field is symmetric about the groove centre. In contrast, the in-plane scattering of a planar SPP can also be strongly altered by the presence of the second, magnetic field anti-symmetric mode as depicted in Figure 1c . This asymmetry gives the second mode a valuable function in modifying the in-plane SPP scattering without affecting the vertical photon–SPP coupling. To realize functional structures that capitalize on the different mode symmetries, we first map out the available scattering responses from grooves with different dimensions. Under normally incident plane wave illumination, photon-SPP coupling can be quantified with a SPP generation cross-section. This cross-section is defined as the total SPP power leaving the groove along the metal surface divided by the incident plane wave intensity, σ = P SPP /Φ. 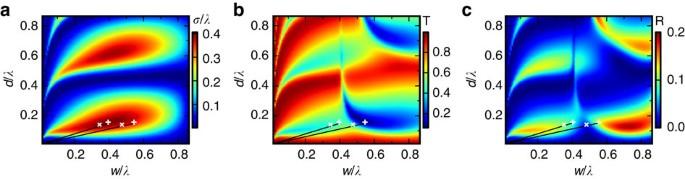Figure 2: Light and SPP scattering response of individual grooves and groove arrays. (a) SPP generation cross-section of a single-gold groove at a wavelength ofλ=700 nm for varying groove width,wand depth,d. (b) SPP transmission across (c) and reflection from a groove. Forw<0.4λ, SPP generation, transmission and reflection are all tied to the fundamental mode resonance within the groove. Forw>0.4λ, excitation of the second mode in the groove decouples the SPP transmission and reflection from SPP generation. The white markers '+' and '×' denote relative groove dimensions for the plasmonic dichroic splitter later on. The black lines indicate paths along which the relative groove dimensions scale with wavelength. In Figure 2a this cross-section is plotted for single-gold grooves of varying dimensions at a wavelength of λ =700 nm. The maxima in the SPP generation cross-section are due to resonances of the fundamental mode within the groove [16] . For the in-plane SPP scattering process, we can quantify the transmission across and reflection from the groove as plotted in Figures 2b and c . For narrow grooves with a width below 0.4 λ , the transmission minima and reflection maxima are also governed by the resonant properties of the fundamental groove mode. This intrinsically ties the in-plane SPP scattering to SPP generation [18] . Around the cutoff of the second mode at a width of 0.4 λ , resonances from the second mode in the groove produce new features in the SPP transmission and reflection [18] , essentially decoupling the in-plane SPP scattering and the SPP generation processes. We for the first time point out that by controlling the groove dimensions, these scattering processes can be independently tuned to realize high-performance and ultracompact photonic devices. Figure 2: Light and SPP scattering response of individual grooves and groove arrays. ( a ) SPP generation cross-section of a single-gold groove at a wavelength of λ =700 nm for varying groove width, w and depth, d . ( b ) SPP transmission across ( c ) and reflection from a groove. For w <0.4 λ , SPP generation, transmission and reflection are all tied to the fundamental mode resonance within the groove. For w >0.4 λ , excitation of the second mode in the groove decouples the SPP transmission and reflection from SPP generation. The white markers '+' and '×' denote relative groove dimensions for the plasmonic dichroic splitter later on. The black lines indicate paths along which the relative groove dimensions scale with wavelength. Full size image Submicron plasmonic dichroic splitter simulation Next, we will show that the unique modal properties of wide (100 nm scale) grooves are very useful for realizing new functionalities. As the groove-scattering behaviour of high-conductivity metals is qualitatively very similar at wavelengths across the visible and near-infrared, the concepts presented have very general applicability. We show that a dichroic (wavelength) splitter can be realized by using two grooves of similar width. The basic idea is that at a specific operating wavelength the groove dimensions can be chosen such that both grooves generate SPPs efficiently, while one transmits SPPs and the other reflects them more efficiently. The reflecting groove will redirect SPPs towards the transmitting groove, causing preferential SPP generation in one direction. At a different wavelength the transmission and reflection roles of the grooves reverse, resulting in dichroic splitting. Our intuitive explanation of the dichroic splitter operation can be made more quantitative by examining the single-groove scattering data presented in Figure 2 . We will consider a somewhat arbitrary case in which we aim to efficiently split light at wavelengths of 650 and 750 nm. Although Figure 2 was calculated at a single wavelength of 700 nm, for the present discussion we assume that it correctly depicts the groove-scattering behaviour at these nearby wavelengths as well. This is reasonable for a qualitative discussion as the metal dispersion only provides secondary corrections to the scattering behaviour. The first requirement for the splitter is to efficiently launch SPPs. Figure 2a shows that high-generation cross-sections can be achieved for groove depths of around 0.15 λ and 0.65 λ , about half a wavelength deeper. At these depths, strong standing wave resonances of the fundamental gap plasmon mode supported by the groove can effectively be driven. These resonances can strongly enhance the coupling of incident free-space photons to SPPs on the metal surface. For the wavelengths of interest the 0.15 λ depth corresponds to a groove depth of about d =100 nm, which is easy to realize in practice. As a second step towards the realization of the dichroic splitter, we need to identify two groove widths that exhibit a strong and opposite wavelength dependence in the transmission of SPPs. To this end, we analyse Figures 2b and c that show how the transmission and reflection behaviour changes with wavelength for specific groove dimensions. Both regions with high groove transmission and reflection can be identified. Particularly sharp features in the SPP transmission behaviour are located at a width around 0.4 λ , right at the cutoff of the second mode. We can take advantage of these features to realize an effective dichroic splitter. Using the graphs, we can show that groove widths, w , of 260 nm and 360 nm make an excellent choice to realize a dichroic splitter for the target wavelengths. For the 650 nm wavelength, these groove widths correspond to w / λ values of 0.4 and 0.55, respectively, as marked by the white plus '+' signs. From Figures 2b and c it can be seen that the wider groove reflects better than it transmits, while the narrower groove transmits better than it reflects. Simulating the scattered fields from a structure in which these two grooves are spaced by 315 nm, we find that SPPs are preferentially generated towards the left with a contrast in power of 3:1, and a total of 70% of the light directly incident on the structure being converted to SPPs ( Fig. 3a ). The groove spacing was chosen using numerical optimization and represents a situation in which the constructive interference of the SPPs launched by the two grooves is maximized. At the longer wavelength, of 750 nm, we find that the behaviour of the same two grooves reverses with the narrower groove w =260 nm=0.35 λ , more effectively reflecting SPPs and the wider groove w =360 nm=0.48 λ , more effectively transmitting. These conditions are depicted by the multiplication '×' signs on Figures 2a–c . The × signs are located on a tie line between the + signs and the origin as we keep the groove dimensions d and w the same and only increase the wavelength. At this longer wavelength, we find that SPPs are preferentially launched towards the right with a contrast of 1:2 and a total of 85% of the light incident on the structure being converted into SPPs ( Fig. 3b ). Although the transmission and reflection magnitudes may seem somewhat low, the transmission and reflection coefficients, being the square root of the former, are significantly higher. After constructive interference, the influence of the transmission and reflection from the grooves is substantial enough to account for the dichroic splitting contrast calculated. From this analysis, it is clear that an ultracompact plasmonic dichroic splitter can be realized by exploiting the interplay between two mode symmetries in each individual groove. 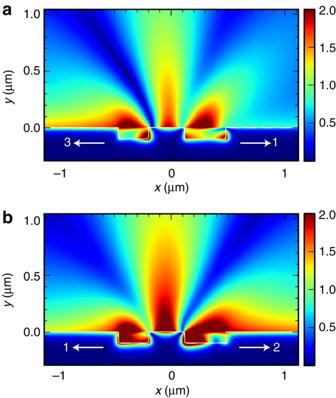Figure 3: Simulated behaviour of a plasmonic dichroic splitter. Two grooves, 260 nm and 360 nm wide, 100 nm deep and 315 nm apart, generate SPPs but exhibit very different SPP transmission and reflection. (a) At a wavelength of 650 nm, directional SPP generation to the left is caused by a transmissive left groove and a reflective right groove. (b) At a wavelength of 750 nm, directional SPP generation to the right is caused by a reflective left groove and a transmissive right groove. Plotted are the magnitudes of the scattered magnetic fields under vertical transverse-magnetic plane wave illumination of amplitude 1. Figure 3: Simulated behaviour of a plasmonic dichroic splitter. Two grooves, 260 nm and 360 nm wide, 100 nm deep and 315 nm apart, generate SPPs but exhibit very different SPP transmission and reflection. ( a ) At a wavelength of 650 nm, directional SPP generation to the left is caused by a transmissive left groove and a reflective right groove. ( b ) At a wavelength of 750 nm, directional SPP generation to the right is caused by a reflective left groove and a transmissive right groove. Plotted are the magnitudes of the scattered magnetic fields under vertical transverse-magnetic plane wave illumination of amplitude 1. Full size image After using the intuitive physical picture described above to identify more-or-less optimum groove dimensions, numerical simulations were used to further optimize the dichroic splitter performance. To this end, we used a transfer-matrix approach accounting for multiple SPP scattering between the grooves (see Methods for details). To facilitate easy fabrication, the depth of both grooves was constrained to the same value. Most grooves naturally exhibit frequencies at which they transition from being reflective to transmissive. The reader may naturally wonder then whether a random pair of asymmetric grooves would also produce similar dichroic behaviour. It is important to realize that multiple conditions must coincidentally be satisfied for the dichroic splitter to function as intended. First, when one groove transitions from reflecting to transmitting when the wavelength is increased, the other groove must undergo the reverse transition. Second, when the grooves transition from reflective to transmissive, both grooves must exhibit a high SPP generation cross-section to maximize the total launched SPP power. Third, to enable broadband dichroic behaviour the frequency range over which the grooves are highly reflective and transmissive must be large. Finally, the spacing between the two grooves must be chosen correctly to allow constructive interference between the SPPs propagating in the desired direction. The first point requires the two grooves to be relatively close in size. The second and third requirements are best satisfied by the relatively wide (that is, low aspect ratio) grooves used here. Wide, shallow grooves are also preferable because they feature lower absorption losses than narrower or deeper grooves, which result in higher SPP generation and reflection. From this discussion, it is clear that randomly selected asymmetric two-groove structures are not very likely to satisfy the multiple conditions necessary for high SPP power and high dichroic splitting ratios. Submicron plasmonic dichroic splitter experiment To experimentally prove the presented concepts, we fabricated a plasmonic dichroic splitter in a gold (Au) film as shown in Figures 1a and 4a . In the centre, the plasmonic dichroic splitter launches SPPs preferentially to the left or right depending on the incident wavelength. Off to the side, two equidistant slits cut through the metal film reconvert the launched SPPs back into photons and enable far-field observation as shown in Figure 1a . The light signal that couples through both observation slits is imaged with a charge coupled device camera. In the experiment, we focused a light beam down to a 3-μm diameter spot onto the two grooves that form the splitter. We determined the spectral dependence of the splitting ratio by integrating the photon counts around each observation slit for wavelengths from 600 nm to 800 nm (see Fig. 4b ). Broadband dichroic behaviour is observed with a 3:1 left:right contrast at 640 nm reversing to a 1:2 left:right contrast at 790 nm around a transition wavelength of 720 nm. 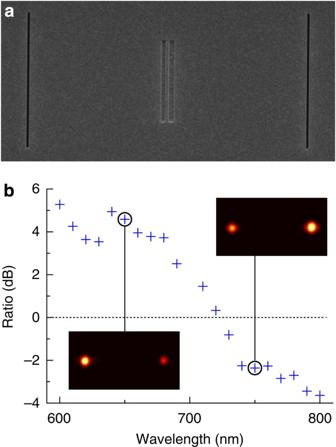Figure 4: Experimental performance of the proposed plasmonic dichroic splitter. (a) Scanning electron microscopy image of the two-groove dichroic splitter with observation slits on the side. The grooves are 280 nm and 380 nm wide and ~110 nm deep, and separated by 300 nm. The observation slits were placed at a 10-μm distance from the splitter and go through the entire metal film. The grooves are 6 μm long and the observation slits are 10 μm long. The structure was fabricated via FIB milling. (b) Spectral dependence of the splitting ratio obtained by integrating the charge coupled device counts at each observation slit for different illumination wavelengths. A 3:1 splitting ratio at short wavelengths reverses to a 1:2 ratio at long wavelengths. Insets show charge coupled device images of the observation slits at 650 nm and 750 nm wavelengths. Images of the observation slits are shown for wavelengths of 650 nm and 750 nm in the insets of Figure 4b . The plasmonic dichroic splitter dimensions and the maximum contrast wavelengths differ slightly from our theoretical prediction because of the mildly sloped sidewalls resulting from FIB and an intermediate aluminium layer used as a milling stop (see Methods). We expect that non-periodic, multi-groove structures will offer larger splitting ratios at the cost of increased device size. Figure 4: Experimental performance of the proposed plasmonic dichroic splitter. ( a ) Scanning electron microscopy image of the two-groove dichroic splitter with observation slits on the side. The grooves are 280 nm and 380 nm wide and ~110 nm deep, and separated by 300 nm. The observation slits were placed at a 10-μm distance from the splitter and go through the entire metal film. The grooves are 6 μm long and the observation slits are 10 μm long. The structure was fabricated via FIB milling. ( b ) Spectral dependence of the splitting ratio obtained by integrating the charge coupled device counts at each observation slit for different illumination wavelengths. A 3:1 splitting ratio at short wavelengths reverses to a 1:2 ratio at long wavelengths. Insets show charge coupled device images of the observation slits at 650 nm and 750 nm wavelengths. Full size image A number of previous plasmonic devices that direct or sort photons from free space have relied on linear and concentric gratings. In one unidirectional SPP coupler design [19] , a slit collects photons and launches SPPs, whereas a separate grating element reflects SPPs into the desired direction. In our current design, the pair of grooves simultaneously functions to collect and direct light. A notable example of plasmonic sorting by Laux et al . [3] , used overlaid concentric or linear gratings to sort light of different wavelengths into apertures. Each grating was designed to collect at one wavelength of light and leave other wavelengths undisturbed. As such, the different structures could clearly be identified with a specific target wavelength. In contrast, our entire dichroic splitter structure effectively interacts with light at both target wavelengths (650 nm and 750 nm). The ability of the grooves in our structure to collect and redirect light at both target wavelengths allows for the realization of such a compact and efficient structure. The field of nanophotonics is using increasingly small metallic and semiconductor nanostructures to control the flow of light. At this time, it is unclear whether wavelength splitting and other optical functions are best accomplished by plasmonic devices, high-index structures or hybrid components. However, it is clear that these materials are preferred as the compactness of an optical device is limited by the range of dielectric constants available to it [1] . It is also clear that one can take advantage of the fact that subwavelength objects support only a very limited number of modes. Near a resonance of such a mode, the scattering behaviour can be greatly enhanced. Moreover, by optically coupling objects together unique scattering responses can be engineered by exploiting strong intermodal interference effects. In this vein, we have shown how the distinct symmetry of groove modes can enable an ultracompact dichroic splitter. The presented advances in manipulating plasmons on patterned surfaces represent another important step towards the realization of the promise of plasmonics as the next chip-scale technology [20] , [21] . Fabrication The patterned metal structures were generated in a metal film on a quartz substrate by FIB. The metal film consisted of a 5-nm Cr adhesion layer, a 186-nm Au layer, a 30-nm aluminium layer and an 80-nm Au layer. The intermediate Al layer in the Au film was used as a slow etch rate FIB stop to control the exact groove depth of the two-groove photon sorter. Measurement To excite SPPs we focused an incident light beam down to a 3-μm diameter onto the plasmonic dichroic splitter. A fraction of the excited SPPs leaked through our equidistant observation slits, and their subsequent far-field radiation was collected through the quartz substrate. Different illumination wavelengths were selected from a Fianium supercontinuum source coupled to an acousto-optic tunable filter and with a single-mode fibre output. The fibre output was first collimated and then focused on the grooves with a 10× 0.26 NA objective. Photons from the observation slit were collected through the quartz substrate with a 50× 0.55 NA objective and imaged with a cooled PIXIS 7520-002 charge coupled device camera. Simulation Simulations performed here rely on the finite difference frequency domain method [22] . The SPP scattering and excitation amplitudes were evaluated from full-field simulations using mode projection [18] , [23] . The dielectric constants of Au were approximated using the Brendal–Borman model [24] . To optimize the dichroic splitter we rely on a modified transfer matrix method [25] . For a general multi-groove structure, we can relate the incident and outgoing SPP amplitudes on each side of the n th groove through the scattering coefficients in equation 1 below. Here we use a n − and a n + to denote the right-propagating SPP amplitudes on the left and right sides of the n th groove and b n − and b n + to denote the left-propagating SPP amplitudes on the left and right sides of the n th groove. The phase of the amplitudes is defined relative to the electric field component perpendicular to the metal–insulator interface. An additional term is introduced to the transfer matrix equation because of SPP generation from vertically incident free-space flux, Φ. t and r are the SPP transmission and reflection coefficients of a groove. S is the right SPP generation coefficient and is defined as the right-propagating SPP amplitude generated on the right side of the groove by an incident flux of Φ=1. From symmetry considerations and our phase convention, the left SPP generation coefficient is given by - S . The total SPP generation cross-section of the groove is then σ =2| S | 2 . The scattering coefficients t , r and S are calculated from finite-difference frequency domain simulations [22] of single grooves using mode projection [18] , [23] and shown in Figure 2 . Furthermore, the SPP amplitudes at neighbouring grooves are related through the known SPP propagation constant, k SPP , and the separation distance, l , as follows. By specifying the incident free-space flux and the incident SPP amplitudes on the first and last grooves, equations 1 and 2 allow us to calculate the SPP amplitudes leaving a multi-groove structure. This simplifies calculating the behaviour of more complex multi-groove structures to the addition and multiplication of 2×2 matrices once the response of a single groove is known. We designed the plasmonic dichroic splitter with these transfer matrix equations by using the sum of the left SPP generation at a wavelength of 650 nm and the right SPP generation at a wavelength of 750 nm as the figure of merit. We found locally optimal structure dimensions following the method of steepest ascent. The transfer matrix method is not exact because we have ignored the free-space waves between the grooves that can scatter back into the SPPs [26] ; however, close to the surface plasmon frequency, this component can be considered a secondary correction. To add a degree of correction for this inaccuracy we found a global optimum by ultimately comparing full-field simulations of our approximate local optima. How to cite this article: Liu J.S.Q. et al . A submicron plasmonic dichroic splitter. Nat. Commun. 2:525 doi: 10.1038/ncomms1537 (2011).